Natural variation inOsMYB8confers diurnal floret opening time divergence betweenindicaandjaponicasubspecies 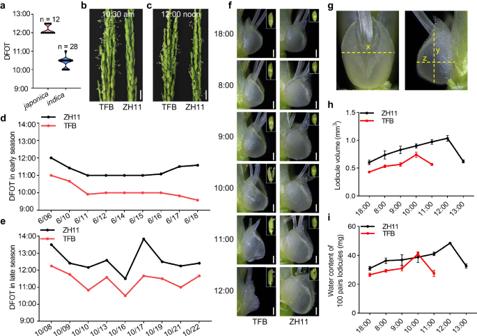Fig. 1: DFOT divergence in rice subspecies. aDiurnal floret opening time (DFOT) ofjaponicacultivars (n= 12 accessions) andindicacultivars (n= 28 accessions) in October 2019 in Guangzhou.b,cComparison of panicles undergoing floret opening in theindicacultivar TFB andjaponicacultivar ZH11 at 10:30 am (b) and 12:00 noon in October 2020 in Guangzhou (c). Scale bars, 1 cm.d,eThe DFOT of TFB and ZH11 in June 2020 in Guangzhou (d) and October 2020 in Guangzhou (e).fLodicule morphology of TFB and ZH11 at different time points in October 2020 in Guangzhou. Scale bars, 250 μm. The boxed areas indicate the corresponding florets. (n= 10 lodicules).gViewing the lodicule as an ellipsoid, its x, y, and z-axes are shown in the diagram.hQuantitative comparison of lodicules volume in ZH11 and TFB at different time points. Lodicule volume was calculated using the ellipsoid volume formula (V = 4πabc/3).a,b, andccorrespond to the semi-axes along the x, y, and z-axes shown in g. Values are means ± SEM. (n= 10 lodicules).iAnalysis of the water content of 100 pairs lodicules of ZH11 and TFB at different time points. Values are means ± SEM. (n= 3 biological replicates). Source data are provided as a Source Data file. The inter-subspecific indica - japonica hybrid rice confer potential higher yield than the widely used indica - indica intra-subspecific hybrid rice. Nevertheless, the utilization of this strong heterosis is currently hindered by asynchronous diurnal floret opening time (DFOT) of indica and japonica parental lines. Here, we identify OsMYB8 as a key regulator of rice DFOT. OsMYB8 induces the transcription of JA-Ile synthetase OsJAR1 , thereby regulating the expression of genes related to cell osmolality and cell wall remodeling in lodicules to promote floret opening. Natural variations of OsMYB8 promoter contribute to its differential expression, thus differential transcription of OsJAR1 and accumulation of JA-Ile in lodicules of indica and japonica subspecies. Furthermore, introgression of the indica haplotype of OsMYB8 into japonica effectively promotes DFOT in japonica . Our findings reveal an OsMYB8 - OsJAR1 module that regulates differential DFOT in indica and japonica , and provide a strategy for breeding early DFOT japonica to facilitate breeding of indica - japonica hybrids. Rice ( Oryza sativa L.) is the preferred major staple crop for over half of the world population (FAO statistical databases, 2022). Historically, several major leaps in rice yield per unit land area have occurred due to improvement of breeding technologies and utilization of advanced cultivars. A major landmark in rice breeding is the utilization of the semi-dwarf gene sd1 (encoding an enzyme essential for gibberellin biosynthesis) and breeding of lodging-resistant rice cultivars in the 1950s, leading to the “first-green revolution” in rice production (average rice yield increased from ~150 kg/mu to 300 kg/mu) [1] . The second landmark in rice breeding is development of hybrid rice in China in the 1970s, led by a group of scientists headed by professor Longping Yuan. Two-hybrid rice breeding technologies, the “three-line” (based on CMS-WA cytoplasmic male sterility) and the “two-line” (based on photoperiod- or thermo-sensitive male sterility) hybrid systems, were developed sequentially in China in the 1970s and 1980s respectively, and are still widely used nowadays [2] , [3] , [4] . Three-line hybrid rice has a yield advantage of ~20–30% over the traditional inbred varieties, and two-line hybrid rice could confer ~5–10% additional yield increase over three-line hybrid rice [5] . To date, the large-scale application of commercial hybrid rice has increased total accumulated rice yield by over 0.6 billion tons, contributing significantly to securing global food supply [6] , [7] . Indica and japonica are two major genetically differentiated ecotypes of Asian cultivated rice. Currently, the majority of hybrid rice is intra-subspecific hybrid rice produced from crosses between indica varieties, with few inter-subspecific hybrid rice produced from crosses between indica and japonica subspecies (China Rice Data Center, https://www.ricedata.cn ). Over the past few decades, yield of intra-subspecific indica hybrid rice has reached a plateau due to the limited genetic diversity of the parental lines [8] . As indica-japonica inter-subspecific hybrid rice has a yield advantage of ~15–30% over the intra-subspecific indica/indica hybrid rice, it is believed that developing more indica-japonica inter-subspecific hybrid rice is an essential route to boost rice production in the future. Nevertheless, production of indica-japonica hybrid rice is currently hindered by several technical bottlenecks, such as hybrid male sterility, prolonged life span, prone to lodging of the hybrids due to exaggerated plant height, and low yield of hybrid seed production. A major reason for low yield of hybrid seed production is asynchronous diurnal floret opening time (DFOT) of the indica and japonica parental lines. During production of indica-japonica inter-subspecific hybrid rice, japonica varieties are often used as the male sterile lines (maternal parent), whereas indica varieties are often used as the pollen donors (parental line). In general, indica rice has an earlier DFOT than japonica rice (average 1–3 h) [9] . This asynchronous DFOT of indica and japonica would severely reduce the efficiency of cross-pollination and large-scale hybrid seed production [10] . Therefore, genetic improvement and synchronization of DFOT of the indica and japonica parental lines are urgently needed for successful commercial production of indica-japonica inter-subspecific hybrid rice seeds. Previous studies have revealed that lodicule, a small scale-like organ lying between the lemma/palea and stamens within the base of florets, plays an important role in controlling DFOT in rice. During floret opening, the lodicule cells absorb water and expand, pushing the lemma and palea apart to drive floret opening. After pollination, lodicule loses water and undergoes programmed cell death, leading to closure of the glumes [10] , [11] , [12] . The opening and closing processes of rice spikelets entail a dynamic change of turgor and osmotic pressure in the parenchymatous cells of the lodicule [13] , [14] , [15] . Mounting evidence indicated that the plant hormone jasmonic acid (JA) plays a key role in regulating floret opening and closure in rice and other monocotyledonous plant species such as wheat and rye [16] , [17] , [18] , [19] . In addition, several recent studies have reported that Diurnal Flower Opening Time 1 ( DFOT1 ) / Early Morning Flowering1 ( EMF1 ), which encodes a DUF642 domain-containing protein, negatively regulates rice DFOT through modulating methylesterification of lodicule cell wall pectin [11] , [20] . Despite the progress made in this field, the genetic basis and molecular mechanisms regulating DFOT in rice, especially the differentiation of DFOT in indica and japonica , have remained essentially unknown. In this study, we identify an R2R3-MYB transcription factor OsMYB8 as a key regulator of asynchronous DFOT by performing a comparative time-course transcriptome analysis of lodicules in indica and japonica . We find that OsMYB8 promotes floret opening in both indica and japonica rice through directly activating the expression of a JA biosynthesis gene OsJAR1 , leading to elevated JA-Ile accumulation and thus altered expression of genes related to cell osmolality and cell wall remodeling in the lodicules. We also reveal that natural variation in the promoter sequences of OsMYB8 confers higher expression level of OsMYB8 in indica , thus higher accumulation of JA-Ile and earlier DFOT in indica as compared to japonica . Finally, we demonstrate that introgression of the indica OsMYB8 allele into japonica rice could confer earlier DFOT in japonica rice. Our study not only provides a significant breakthrough into the understanding of the genetic network regulating asynchronous DFOT of indica and japonica rice but also provides effective genetic resources for genetic improvement of rice DFOT to facilitate hybrid breeding between indica and japonica subspecies. Diurnal floret opening time divergence in rice subspecies To investigate the genetic variation for the DFOT trait in rice, we collected a rice diversity panel, including 12 japonica and 28 indica cultivars (Supplementary Data 1 ), and compared their DFOT in October 2019 in Guangzhou (Longitude, 113.27°; Latitude, 23.13°). The results showed that the indica cultivars exhibited the peak opening time at around 10:00–11:00 am, whereas the japonica cultivars had peak opening time at approximately 12:00–12:30 noon, indicating that the DFOT of indica cultivars was significantly earlier than that of japonica cultivars (Fig. 1a , Supplementary Data 1 ). Subsequently, the DFOT trait of a typical indica cultivar TianFengB (TFB) and a typical japonica cultivar ZhongHua11 (ZH11) was further analyzed in the early (June) and late (October) growing seasons of 2020 in Guangzhou. As expected, the DFOT of TFB was 1–2 h earlier than that of ZH11 in both the early and late seasons (Fig. 1b–e ). Meanwhile, we carefully recorded the size and morphology of the lodicules of TFB and ZH11 at different time points under a stereomicroscope. The results showed that the lodicules of TFB swelled and reached the maximum size by 10:00 am, while the lodicules of ZH11 displayed a delay in swelling and did not reach the maximum size until 12:00 noon (Fig. 1f–h ). Measurement of water content in the lodicules of TFB and ZH11 at different time points revealed a gradual increase of water content as the floret opening time approaching. Water content reached the highest at 10:00 am in the lodicules of TFB, but did not reach the highest until 12:00 noon in ZH11 (Fig. 1i ). Taken together, these results indicate that the indica cultivars exhibit earlier DFOT than japonica cultivars, which could be attributed to advanced swelling of the lodicules in indica cultivars. Fig. 1: DFOT divergence in rice subspecies. a Diurnal floret opening time (DFOT) of japonica cultivars ( n = 12 accessions) and indica cultivars ( n = 28 accessions) in October 2019 in Guangzhou. b , c Comparison of panicles undergoing floret opening in the indica cultivar TFB and japonica cultivar ZH11 at 10:30 am ( b ) and 12:00 noon in October 2020 in Guangzhou ( c ). Scale bars, 1 cm. d , e The DFOT of TFB and ZH11 in June 2020 in Guangzhou ( d ) and October 2020 in Guangzhou ( e ). f Lodicule morphology of TFB and ZH11 at different time points in October 2020 in Guangzhou. Scale bars, 250 μm. The boxed areas indicate the corresponding florets. 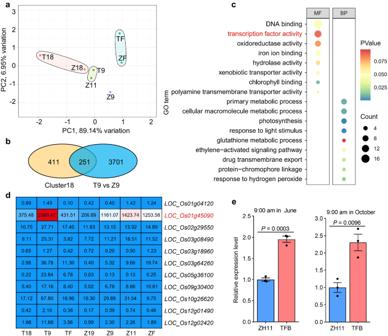Fig. 2: Identification ofOsMYB8by comparative transcriptomic analysis of lodicules betweenindicaandjaponica. aPrincipal component analysis (PCA) of the transcriptome datasets of lodicules between TFB and ZH11 at different time points. T18 and Z18 indicate 18:00 the day before floret opening; T9 and Z9 indicate 9:00 am (1 h and 3 h before floret opening in TFB and ZH11, respectively); Z11 indicate 11:00 am (1 h before opening in ZH11); TF and ZF indicate the time undergoing peak floret opening time (~10:00 am in TFB; ~12:00 noon in ZH11).bVenn Diagram showing the number of overlapping genes between the Cluster18 genes and up-regulated DEGs from T9 vs Z9.cGene Ontology (GO) enrichment analysis of 251 overlap genes in (b). MF indicates molecular function, BP indicates biological process. The term of “transcription factor activity” is highlighted in red.dExpression analysis of 11 transcription factors selected through GO analysis in (c). The numbers in the heatmap represent the average FPKM values.eReverse transcriptional quantitative PCR (RT-qPCR) analysis ofOsMYB8expression level in the lodicules of TFB and ZH11 at 9:00 am in June and October in 2021. Values are mean ± SEM. (n= 3 biological replicates). Significance is evaluated by the two-sided Student’st-test at each time point, andPvalues are indicated. Source data are provided as a Source Data file. ( n = 10 lodicules). g Viewing the lodicule as an ellipsoid, its x, y, and z-axes are shown in the diagram. h Quantitative comparison of lodicules volume in ZH11 and TFB at different time points. Lodicule volume was calculated using the ellipsoid volume formula (V = 4πabc/3). a , b , and c correspond to the semi-axes along the x, y, and z-axes shown in g. Values are means ± SEM. ( n = 10 lodicules). i Analysis of the water content of 100 pairs lodicules of ZH11 and TFB at different time points. Values are means ± SEM. ( n = 3 biological replicates). Source data are provided as a Source Data file. Full size image Identification of OsMYB8 as a key regulator of differential DFOT in indica and japonica To explore the molecular basis underlying the differential lodicule swelling in indica and japonica , we performed a comprehensive comparative RNA-seq analysis of the lodicules of TFB and ZH11 at different time points, including 18:00 the day before floret opening (T18 in TFB, Z18 in ZH11), 3 h before opening in ZH11 (Z9, ~9:00 am), 1 h before opening (T9, ~9:00 am in TFB; Z11, ~11:00 am in ZH11) and undergoing peak floret opening time (TF, ~10:00 am in TFB; ZF, ~12:00 noon in ZH11) (Supplementary Fig. 1a, b ). Correlation analysis of biological replicates from each time point showed very high correlation coefficients ( R 2 ≥ 0.90; Supplementary Fig. 1c ). Thus, we calculated the average FPKM value of the replicates as the gene expression level for each sample. We further performed pairwise differential gene expression analyses between two consecutive time points and identified 6102 differentially expressed genes (DEGs) between T9 vs. T18, 6326 DEGs between TF vs. T9, 7164 DEGs between Z9 vs. Z18, 2972 DEGs between Z11 vs. Z9, 7012 DEGs between ZF vs. Z11 and 7430 DEGs between T9 vs. Z9 ( P -value < 0.05, absolute log 2 FC (fold change) ≥ 1; Supplementary Fig. 1d ; Supplementary Data 2 ). Gene Ontology (GO) term enrichment analysis revealed that biological processes and molecular pathways related to cell osmolality and cell wall remodeling, such as sugar transport, water channel activity, JA synthesis and signaling, calcium signaling and ethylene signaling were enriched in one or more datasets (Supplementary Fig. 2 ). Principal component analysis (PCA) showed that the dataset of T18 was grouped together with that of Z18. Likewise, the dataset of TF was grouped together with that of ZF (Fig. 2a ). In congruent with earlier DFOT in TFB, the T9 time point was grouped together with Z11 but not Z9, suggesting that transcriptional activities related to floret opening process are advanced in TFB, compared to ZH11 (Fig. 2a ). Fig. 2: Identification of OsMYB8 by comparative transcriptomic analysis of lodicules between indica and japonica . a Principal component analysis (PCA) of the transcriptome datasets of lodicules between TFB and ZH11 at different time points. T18 and Z18 indicate 18:00 the day before floret opening; T9 and Z9 indicate 9:00 am (1 h and 3 h before floret opening in TFB and ZH11, respectively); Z11 indicate 11:00 am (1 h before opening in ZH11); TF and ZF indicate the time undergoing peak floret opening time (~10:00 am in TFB; ~12:00 noon in ZH11). b Venn Diagram showing the number of overlapping genes between the Cluster18 genes and up-regulated DEGs from T9 vs Z9. c Gene Ontology (GO) enrichment analysis of 251 overlap genes in ( b ). MF indicates molecular function, BP indicates biological process. The term of “transcription factor activity” is highlighted in red. d Expression analysis of 11 transcription factors selected through GO analysis in ( c ). The numbers in the heatmap represent the average FPKM values. e Reverse transcriptional quantitative PCR (RT-qPCR) analysis of OsMYB8 expression level in the lodicules of TFB and ZH11 at 9:00 am in June and October in 2021. Values are mean ± SEM. ( n = 3 biological replicates). Significance is evaluated by the two-sided Student’s t -test at each time point, and P values are indicated. Source data are provided as a Source Data file. Full size image Considering that the time point of 1 h before opening is the crucial stage for floret opening [10] , [21] , we speculated that genes responsible for differentiated DFOT in indica and japonica might show characteristic expressional changes in T9 and Z11, and likely be up-regulated in the datasets of T9 vs. Z9. Therefore, we first performed k-means clustering analysis of all expressed genes and identified a total of 20 clusters with distinct gene expression patterns (Supplementary Fig. 1e ). Among them, the Cluster18 genes showing peak expression at T9 and Z11 were selected for further detailed analyses. Next, we performed an overlap analysis of Cluster18 genes with up-regulated DEGs of T9 vs. Z9. A total of 251 overlapping genes were identified (Fig. 2b ). GO term analysis revealed an enrichment of DNA binding and transcription factor activity (Fig. 2c ). We further noted that among the 11 overlapping genes encoding transcription factors, LOC_Os01g45090 ( OsMYB8 ), encoding an R2R3-MYB transcription factor, exhibited the highest expression level and was gradually up-regulated in the lodicules before floret opening (Fig. 2d ). Neighbor-joining tree analysis showed that OsMYB8 is homologous to AtMYB21 / 24 , which are involved in JA signaling and regulating stamen development in Arabidopsis [22] (Supplementary Fig. 3 ). The RiceXPro data and reverse transcriptional quantitative PCR (RT-qPCR) analyses showed that OsMYB8 was preferentially expressed in lemma, palea, stamen, stigma, and lodicule, but with low expression level in root, stem, leaf, and young panicle (Supplementary Fig. 4a, b ). Histochemical staining analysis of transgenic lines expressing the pOsMYB8::GUS (β-glucuronidase) reporter gene also revealed a similar expression pattern (Supplementary Fig. 4c ). RT-qPCR analysis showed that the expression level of OsMYB8 was lower in the lodicules of TFB and ZH11 at the day before floret opening, and then gradually increased towards opening time, and decreased thereafter. Additionally, we found that the expression level of OsMYB8 in indica lodicules was significantly higher than that in japonica lodicules before floret opening (Supplementary Fig. 5 ). Moreover, RT-qPCR analysis verified that the expression levels of OsMYB8 in the lodicules of TFB at 9:00 am (the time before floret opening) were about 2-fold of that in ZH11 at the same time points (Fig. 2e ). These observations together suggest that the elevated expression level and an earlier peak expression time of OsMYB8 in TFB compared with that in ZH11 may contribute to the earlier floret opening time in indica varieties. Thus, we selected OsMYB8 as a candidate gene regulating the differentiated DFOT in indica and japonica subspecies. OsMYB8 promotes floret opening in rice To explore the role of OsMYB8 in DFOT regulation, we knocked out the OsMYB8 gene in both ZH11 and TFB backgrounds using the CRISPR/Cas9 technology. Two verified independent OsMYB8 knockout lines in ZH11 ( Osmyb8 ZH #1 and Osmyb8 ZH #2 ) and TFB background ( Osmyb8 TF #1 and Osmyb8 TF #2 ) were selected for detailed phenotypic analysis (Fig. 3a , Supplementary Fig. 6 ). The florets of ZH11 started opening at around 10:30 am, and achieved peak opening time by 11:30 am, whereas the Osmyb8 ZH mutants did not achieve peak opening time until 12:00 noon, about 0.5 h later than ZH11 (Fig. 3b, c ). Similarly, the peak opening time of the Osmyb8 TF mutants was about 1 h later than TFB (Fig. 3e, f ). In addition, given that OsMYB8 showed higher expression level in TFB than in ZH11, we also generated two transgenic lines expressing OsMYB8 of TFB (including the coding sequence and 2-kb upstream promoter sequence) in the ZH11 background ( OsMYB8 TF /ZH11 #1 and OsMYB8 TF /ZH11 #2 ) (Fig. 3h, i ). As shown in Fig. 3j , the peak opening time of the OsMYB8 TF /ZH11 plants occurred ~0.5–1 h earlier than ZH11 (Fig. 3j, k ). The daily number of opening florets of both the Osmyb8 mutants and OsMYB8 TF /ZH11 lines was comparable to that of the wild-type plants (Fig. 3d, g, l ). Additionally, both the OsMYB8 knockout lines in ZH11 and TFB backgrounds exhibited normal spikelet and stamen development, and their anthers also dehisced normally (Supplementary Fig. 7a–c ). Besides, I 2 -KI (potassium iodide) solution staining experiments showed that the pollen fertility of the Osmyb8 mutants were comparable to that of the WT plants (Supplementary Fig. 7d, e ). Moreover, seed setting rates of Osmyb8 ZH #1 and Osmyb8 ZH #2 were comparable to ZH11, while Osmyb8 TF #1 and Osmyb8 TF #2 showed slightly lower seed setting rates compared to TFB (Supplementary Fig. 7f ). These results demonstrated that OsMYB8 primarily acts to promote rice floret opening but confer minimal influence on the pollen development and spikelet fertility. Fig. 3: OsMYB8 positively regulates rice DFOT. a Creation of the Osmyb8 mutants using the CRISPR/Cas9 genome editing approach. Osmyb8 mutants in ZH11 and TFB backgrounds were named as Osmyb8 ZH and Osmyb8 TF respectively. The upper panel shows a schematic diagram of the OsMYB8 gene bearing the CRISPR/Cas9 target site. The mutation site was indicated in red. b , e , j Comparison of panicles in ZH11 and Osmyb8 ZH mutants at 11:30 am ( b ) TFB and Osmyb8 TF mutants at 10:00 am ( e ) ZH11 and OsMYB8 TF /ZH11 lines at 10:00 am in June 2021 in Guangzhou ( j ). Scale bars, 1 cm. c , f , k Number of opened florets per panicle in ZH11 and Osmyb8 ZH mutants ( c ), TFB and Osmyb8 TF mutants ( f ), and ZH11 and OsMYB8 TF /ZH11 lines ( k ) at different time points of the day in June 2021 in Guangzhou. Values are means ± SEM. ( n = 8 panicles). d , g , l Number of opened florets in ZH11 and Osmyb8 ZH mutants ( d ), TFB and Osmyb8 TF mutants ( g ), and ZH11 and OsMYB8 TF /ZH11 lines ( l ) at different days after heading in June 2021 in Guangzhou. Values are means ± SEM. ( n = 10 panicles). h Schematic diagram of the vector structure used for constructing OsMYB8 TF /ZH11 transgenic plants. i RT-qPCR analysis of OsMYB8 transcripts levels in the lodicules of the OsMYB8 TF /ZH11 transgenic lines. ZH11 was used as a negative control. Values are means ± SEM. ( n = 3 biological replicates). Significance is evaluated by the two-sided Student’s t -test, and P values are indicated. Source data are provided as a Source Data file. Full size image Identification of the genome-wide direct targets of OsMYB8 Consistent with OsMYB8 encoding an R2R3-MYB transcription factor, the OsMYB8-GFP fusion protein was localized to the nucleus in rice protoplasts (Fig. 4a ). Moreover, transcriptional activity analysis of OsMYB8 in yeast revealed that OsMYB8 is a transcriptional activator and the activation domain is located at its C-terminus (Fig. 4b ). Fig. 4: Identification of the genome-wide direct targets of OsMYB8. a Nuclear localization of OsMYB8-GFP in rice protoplasts. D53-mCherry was used as a nuclear marker. Scale bars, 20 μm. b Yeast two-hybrid assay showing the transcriptional activity of OsMYB8. Left is the diagrams of full-length and truncated OsMYB8 proteins, which were fused with the DNA-binding domain (BD). c The core binding motif of OsMYB8 protein identified using MEME-ChIP. d Venn diagrams showing a comparison of DAP-seq binding genes with the identified DEGs in Osmyb8 mutants by RNA-seq. e GO enrichment analysis of 345 overlap genes in ( d ). MF indicates molecular function, BP indicates biological process. f ChIP-qPCR analysis showing that OsMYB8 binds to the OsJAR1 promoter in vivo. The upper panel is a diagram of OsJAR1 promoter with the indicated regions used for detection by ChIP-qPCR. The red lines indicate the position of “TTHGGY” motifs in the OsJAR1 promoter regions. Immunoprecipitation was performed with anti-GFP antibody, ZH11 was used as a negative control. ( n = 3 technical replicates). g EMSA assay showing that GST-OsMYB8 recombinant protein directly binds to the “TTHGGY” motif-containing regions of the OsJAR1 promoter. Unlabeled probes were used as competitors. GST was used as a negative control. h Transient dual-LUC assay showing that OsMYB8 induces the transcriptions of OsJAR1 promoter in rice protoplasts. The upper panel is diagrams of various constructs used in the transient expression assay. The expression level of REN was used as an internal control. The LUC/REN ratio represents the relative activity of the OsJAR1 promoter. ( n = 3 technical replicates). The Values in ( f ) and ( h ) are means ± SEM. Significance is evaluated by the two-sided Student’s t -test, and P values are indicated. The subcellular localization experiments in ( a ) and the EMSA experiments in ( g ) were independently repeated three times with similar results. Source data are provided as a Source Data file. Full size image To identify the direct downstream targets of OsMYB8, we first performed DNA affinity purification sequencing (DAP-seq) to unravel its genome-wide binding sites. Purified recombinant GST-OsMYB8 fusion protein (expressed in E. coli ) was used to affinity purify the sheared genomic DNA of 14-day old ZH11 seedlings, followed by deep sequencing (Supplementary Fig. 8a ). In total, 27,764 binding peaks located within the regulatory regions of 20,832 genes were detected (Supplementary Data 3 ), 70.74% of which were distributed in the promoter or intergenic regions, 13.26% and 11.82% were in the exon and the intron regions respectively, while 4.18% was in the 5′UTR and 3′UTR regions (Supplementary Fig. 8b ). By using the MEME Suite, a representative DNA binding motif of MYB proteins with a core sequence of “TTHGGY” (H indicates A/T/G, Y indicates T/C) was significantly enriched among the OsMYB8 binding regions [23] (Fig. 4c ). To verify the reliability of our DAP-seq result, we randomly selected 3 putative target genes, and further carried out electrophoretic mobility shift assays (EMSAs) using native promoter probes harboring the wild-type “TTHGGY” motif or its mutated forms “TTHAAY”. The results showed that OsMYB8 could directly bind to the native promoter probes, whereas mutations in the “TTHGGY” motif largely abolished the binding of OsMYB8 (Supplementary Fig. 8c ), thus confirming that OsMYB8 could directly bind to the “TTHGGY” motif. To narrow down the potential direct targets of OsMYB8 for regulating rice DFOT, we performed RNA-seq of the lodicules of TFB and Osmyb8 TF collected at 9:00 am or lodicules of ZH11 and Osmyb8 ZH collected at 10:00 am. Correlation analysis showed very high correlation coefficients within three biological replicates for each group (Supplementary Fig. 8d ). Among them, 2629 DEGs were identified between TFB vs. Osmyb8 TF , and 4419 DEGs were identified between ZH11 vs. Osmyb8 ZH , respectively ( P -value < 0.05, absolute log 2 FC ≥ 1; Supplementary Fig. 8e , Supplementary Data 4 , 5 ). By overlapping analysis of the DEGs and the OsMYB8 binding genes, we identified 345 potential genes that were differentially expressed in Osmyb8 lodicules and directly bound by OsMYB8 (Fig. 4d ). GO term analysis revealed significant enrichment of several molecular functions known to be related to lodicule swelling and closure, such as cell wall modification and regulation of JA-mediated signaling pathway (Fig. 4e , Supplementary Data 6 ). Among them, the OsJAR1 gene, which encodes an enzyme essential for the conversion of JA to active JA (JA-Ile) [24] , was down-regulated in the lodicules of the Osmyb8 mutants, but up-regulated in the lodicules of the OsMYB8 TF /ZH11 lines (Supplementary Fig. 9a–c ). RT-qPCR analysis revealed that similar to OsMYB8 , the expression level of OsJAR1 in the lodicules of TFB and ZH11 increases as the floret opening time approaches (Supplementary Fig. 9d ). To verify that OsJAR1 is a direct target of OsMYB8, we analyzed the promoter region of OsJAR1 , and identified a set of OsMYB8 binding motifs (TTHGGY) in the 2-kb region upstream of the transcription start site (Fig. 4f ). To examine the binding capacity of OsMYB8 to the OsJAR1 promoter in vivo, we generated two transgenic lines with stable expression of OsMYB8-GFP driven by the native OsMYB8 promoter of TFB (Supplementary Fig. 10a–c ). We also found that the OsMYB8-GFP lines exhibited about 1 h earlier DFOT than ZH11 (Supplementary Fig. 10d, e ), suggesting that the OsMYB8-GFP fusion protein is biologically functional. ChIP-qPCR assays using florets of the OsMYB8-GFP#2 transgenic line showed that anti-GFP antibody could specifically precipitate the P1 and P3 fragments containing the OsMYB8 binding motif in the OsJAR1 promoter (Fig. 4f ). EMSAs also demonstrated that GST-OsMYB8 could directly bind to the P1 and P3 fragments of the OsJAR1 promoter (Fig. 4g ). In addition, transient expression assay in rice protoplasts showed that LUC expression driven by the native OsJAR1 promoter was increased significantly when the reporter was co-transformed with the OsMYB8 effector in rice protoplasts (Fig. 4h ). Taken together, our findings suggest that OsMYB8 directly activates OsJAR1 transcription. OsMYB8 genetically acts upstream of OsJAR1 to regulate rice DFOT To test whether OsJAR1 regulates rice DFOT, we performed targeted mutagenesis of OsJAR1 in the ZH11 background using the CRISPR/Cas9 technology. Two independent knockout lines ( Osjar1#1 and Osjar1#2 ) were obtained for phenotypic analysis (Fig. 5a ). We counted the number of opened florets at different time points of ZH11 and Osjar1 mutants in June 2022 in Guangzhou, and found that in contrast to ZH11, which had a peak DFOT at around 11:30 am, the Osjar1 mutants displayed a scattered floret opening phenotype (random floret opening throughout the day), indicating that OsJAR1 is required for proper floret opening (Fig. 5b, c ). As expected, measurement of JA-Ile in the lodicules of ZH11, Osjar1 mutant and Osmyb8 ZH showed that the JA-Ile content in the lodicules of Osjar1 and Osmyb8 ZH mutant was significantly lower than that of ZH11 (Fig. 5d ). In contrast, the JA-Ile content of OsMYB8 TF /ZH11 was significantly higher than that of ZH11 (Fig. 5e ). These data together suggest that OsMYB8 regulates JA-Ile content in lodicules to promote floret opening in rice. Fig. 5: OsJAR1 influences JA-Ile content in lodicule to regulate rice DFOT. a Creation of the Osjar1 mutants in ZH11 background using the CRISPR/Cas9 genome editing approach. The mutation site was indicated in red. b Comparison of panicles in ZH11 and Osjar1 mutants at 11:30 am in June 2022 in Guangzhou. Scale bars, 1 cm. c Number of opened florets per panicle in ZH11 and Osjar1 mutants at different time points of the day. Values are mean ± SEM. ( n = 10 panicles). d , e JA-Ile content in lodicules at 10:00 am of ZH11, Osjar1, and Osmyb8 ZH ( d ) at 9:00 am of ZH11 and OsMYB8 TF /ZH11( e ). Values are mean ± SEM. ( n =  3 biological replicates). Significance is evaluated by the two-sided Student’s t -test, and P values are indicated. f Schematic diagram of the vector structure used for constructing OsJAR1 com materials. The pOsMYB8 TF means the promoter was amplified from TFB. g Relative expression level of OsJAR1 in the lodicules of ZH11, OsJAR1 com and Osmyb8 ZH . Values are means ± SEM. ( n = 3 biological replicates). Letters above the bars indicate significant differences ( P < 0.05), as evaluated by one-way ANOVA with Tukey’s multiple comparisons test. h , j Comparison of panicles in ZH11, OsJAR1 com and Osmyb8 ZH at 11:30 am in June 2022 in Guangzhou ( h ) and in ZH11, OsMYB8 TF /ZH11, OsMYB8 TF / Osjar1 and Osjar1 at 12:00 noon in October 2022 in Guangzhou ( j ). Scale bars, 1 cm. i Number of opened florets in ZH11, OsJAR1 com , and Osmyb8 ZH at different time points of the day in June 2022 in Guangzhou. Values are mean ± SEM. ( n = 10 panicles). k Number of opened florets in ZH11, OsMYB8 TF /ZH11, OsMYB8 TF / Osjar1, and Osjar1 at different time points of the day in October 2022 in Guangzhou. Values are mean ± SEM. ( n = 10 panicles). Source data are provided as a Source Data file. Full size image To further determine the genetic relationship between OsJAR1 and OsMYB8 , we introduced the OsJAR1 coding sequence driven by the OsMYB8 promoter of TFB (which possesses high transcriptional activity in lodicules, Fig. 2d ) into the Osmyb8 ZH mutant background (Fig. 5f ). Two independent transgenic lines ( OsJAR1 com #1 and OsJAR1 com #2 ) with higher OsJAR1 expression level in lodicules than that of ZH11 and Osmyb8 ZH exhibited an intermediate peak DFOT between ZH11 and Osmyb8 ZH (Fig. 5g–i ), suggesting that up-regulation of OsJAR1 expression could partially complement the delayed DFOT of Osmyb8 ZH . Moreover, we generated OsMYB8 TF / Osjar1 line by crossing OsMYB8 TF /ZH11 with an Osjar1 line and found that the OsMYB8 TF /Osjar1 line displayed a scattered floret opening phenotype, similar to Osjar1 (Fig. 5j, k ). These observations support the placement of OsJAR1 downstream of OsMYB8 to regulate DFOT in rice. As genes related to cell osmolality and cell wall remodeling play a predominant role in DFOT regulation [10] , [21] (Supplementary Fig. 2 ), we next tested whether dysfunction of OsJAR1 could influence their expressions. As expected, we found that a series of differentially expressed genes associated with carbohydrate metabolic process, sugar transport, cell wall organization, and water channel activity showed altered expression in the transcriptome data of TFB vs. Osmyb8 TF and ZH11 vs. Osmyb8 ZH (Supplementary Fig. 11a ), and most of the DEGs were down-regulated in lodicules of both Osmyb8 TF and Osmyb8 ZH . Remarkably, four Pectin Methylesterase genes ( OsPME12/22/23/29 ) were up-regulated, in line with the potential negative role of this gene family in DFOT regulation [11] . We further performed RT-qPCR analyses to examine the expression changes of these genes in the lodicules of the Osjar1 mutants. As expected, a large portion of genes exhibited similar changes to that of the Osmyb8 mutants. For example, expression of OsAmy2 , Os4BGlu , OsSWEET11/15 , OsEXPB7 , OsXTH16 , OsPG17 and OsNIP1;1 was significantly decreased, while expression of OsPME23/29 was significantly increased (Supplementary Fig. 11b, c ). We further analyzed soluble sugar content in the lodicules of ZH11 and Osmyb8 ZH collected at 10:00 am, and the result showed that the levels of sucrose, fructose and total soluble sugars were decreased in the lodicules of Osmyb8 ZH (Supplementary Fig. 12 ). These results suggest that OsMYB8-OsJAR1 module likely influence floret opening by modulating the expression of genes related to lodicule hydration and expansion. Natural variation in OsMYB8 promoter confers DFOT divergence in japonica and indica To look for the natural variation underlying differential expression of OsMYB8 in indica and japonica rice, we conducted sequence analysis of the coding region and 2-kb promoter sequences of OsMYB8 between TFB and ZH11. The results showed that there are six SNPs (−1176, −1244, −1286, −1469, −1550 and −1871) in the promoter and one synonymous SNP in the coding region (Fig. 6a ). Based on the six SNPs, we performed haplotype analysis of the OsMYB8 2-kb promoter using 1973 indica ( Ind ), 767 temperate japonica ( TeJ ), 504 tropical japonica ( TrJ ), and 269 Aus [25] (Supplementary Data 7 ). A total of three haplotypes (Hap1–3) was identified in these rice accessions. Hap1 and Hap2 differed in six SNPs, while Hap3 differed from Hap1 at four SNPs (−1286, −1469, −1550, and −1871), and Hap2 at two SNPs (−1176 and −1244) (Fig. 6a ). Hap1 was mainly present in the Ind accessions (including TFB). In contrast, 671 out of 767 (~88.0%) TeJ accessions (including ZH11) carried Hap2. Hap3 was mostly detected in Ind , TrJ, and Aus (Fig. 6b ). To investigate whether OsMYB8 has undergone selection during rice domestication, we surveyed the nucleotide diversity (π) across the OsMYB8 genomic region using 295 Ind and 91 TeJ from a rice core collection [26] and 185 O. rufipogon (Ruf ) [27] (Supplementary Data 8 ). The nucleotide diversity of the OsMYB8 2-kb promoter region was extremely low in Ind (π = 0.00074) and TeJ (π = 0.00076), as compared with that of Ruf (π = 0.0053), and was also much lower than that of the whole genome of O. sativa (π = 0.0024) [28] (Fig. 6c , Supplementary Data 9 ). Meanwhile, the fixation index (F ST ) value around OsMYB8 exhibited a higher level of differentiation between the Ind and TeJ populations ( Ind _ TeJ ) (Fig. 6d , Supplementary Data 10 ). These results indicate that OsMYB8 has undergone divergent selection in the indica and japonica subspecies. Fig. 6: Natural variation in OsMYB8 promoter confers DFOT divergence in japonica and indica . a Haplotype analysis of OsMYB8 promoter in the 3513 rice germplasms. Nucleotide variations in the 2-kb promoter of OsMYB8 were shown. b Distribution frequency of the three OsMYB8 haplotypes in diverse Asian cultivated rice accession. The haplotype with the largest number was highlighted in red. c Nucleotide diversity (π) of a 100-kb genomic region surrounding OsMYB8 in the indica ( Ind ), temperate japonica ( TeJ ) and O. rufipogon ( Ruf ). The regions (Chr1: 25,590,725–25,592,725) between two black vertical lines indicates the position of OsMYB8 promoter. d F ST values of TeJ _ Ind , Ruf _ TeJ , and Ruf _ Ind in a 100-kb genomic region surrounding OsMYB8 . The region (Chr1: 25,590,725–25,592,725) between two black vertical lines indicates the position of OsMYB8 promoter. e The DFOT of the rice accessions with Hap1 and Hap2 in May 2022 in Guangzhou. ( n = 30 accessions). f Relative expression levels of OsMYB8 in lodicules of the rice accessions with Hap1 and Hap2, respectively. ( n = 10 accessions). g JA-Ile content in TFB and ZH11 lodicules at 9:00 am. ( n = 3 biological replicates). h Transient dual-luciferase assays showing the transcriptional activity of pOsMYB8 Hap1 and pOsMYB8 Hap2 in rice protoplasts. ( n = 3 technical replicates). The values in f – h are shown as mean ± SEM. Significance is evaluated by the two-sided Student’s t- test, and P values are indicated. i Relative expression levels of OsMYB8 in lodicules of ZH11, OsMYB8 TF / Osmyb8 ZH transgenic lines and the Osmyb8 ZH mutant. Values are mean ± SEM. ( n = 3 biological replicates). Letters above the bars indicate significant differences ( P < 0.05), as evaluated by one-way ANOVA with Tukey’s multiple comparisons test. j Comparison of panicles in ZH11, OsMYB8 TF / Osmyb8 ZH transgenic lines and the Osmyb8 ZH mutant at 11:30 am in October 2022 in Guangzhou. Scale bars, 1 cm. k Number of opened florets in ZH11, OsMYB8 TF / Osmyb8 ZH transgenic lines, and the Osmyb8 ZH mutant at different time points of the day in October 2022 in Guangzhou. Values are mean ± SEM. ( n = 10 panicles). Source data are provided as a Source Data file. Full size image To further evaluate the functional difference between OsMYB8 Hap1 and OsMYB8 Hap2 , we analyzed dozens of accessions with Hap1 and Hap2, respectively (Supplementary Data 8 ). We found that the Hap1-carrying accessions exhibited earlier DOFT compared to the Hap2-carrying accessions (Fig. 6e ). Furthermore, the Hap1-carrying accessions showed higher levels of OsMYB8 gene expression and JA-Ile level (Fig. 6f, g ). Moreover, transient transcriptional activation experiments showed that the OsMYB8 Hap1 promoter possessed higher transcriptional activity than the OsMYB8 Hap2 promoter in rice protoplast (Fig. 6h ). These findings suggest that the sequence variations between Hap1 and Hap2 might cause differential expression of the OsMYB8 , thus conferring earlier DFOT in the Hap1-carrying varieties as compared to the Hap2-carrying varieties. To consolidate this notion, we introduced the TFB OsMYB8 allele ( OsMYB8 TF ) containing the 2-kb promoter and intact coding region into the Osmyb8 ZH mutant to generate complementary plants. Two independent transgenic lines with single copy insertion of OsMYB8 TF ( OsMYB8 TF / Osmyb8 ZH #1 , OsMYB8 TF / Osmyb8 ZH #2 ) were selected to be further analyzed (Supplementary Fig. 13 ). RT-qPCR analysis showed that the expression levels of OsMYB8 in lodicules of OsMYB8 TF / Osmyb8 ZH plants were about 2-fold that of ZH11 and Osmyb8 ZH mutant (Fig. 6i ), similar to the expression difference of OsMYB8 between TFB and ZH11 (Fig. 2d, e ). Consistently, the expression level of OsJAR1 was higher in OsMYB8 TF / Osmyb8 ZH than in ZH11 and the Osmyb8 ZH mutant, and the JA-Ile content in the lodicules of OsMYB8 TF / Osmyb8 ZH was significantly higher than that of ZH11 (Supplementary Fig. 14 ). Phenotypic analysis showed that the OsMYB8 TF / Osmyb8 ZH plants exhibited about 0.5 and 1 h earlier DFOT than ZH11 and the Osmyb8 ZH mutant, respectively (Fig. 6j, k ). These results together support the notion that the natural variation in the OsMYB8 promoter contributes to the differential expression of OsMYB8 , and thus divergence of DFOT in indica and japonica subspecies. Potential breeding utilization of OsMYB8 Hap1 in DFOT improvement of japonica varieties The asynchronous DFOT of indica and japonica could severely reduce the efficiency of cross-pollination and large-scale hybrid seed production, causing high price of the hybrid seeds. To evaluate the breeding potential of the OsMYB8 Hap1 allele in DFOT improvement of japonica varieties, we introduced the TFB allele of OsMYB8 into ZH11 through backcrossing and marker-assisted selection. The near-isogenic line (NIL) NIL TFB with the introgressed OsMYB8 TFB allele in ZH11 background was selected from BC 4 F 3 plants. We also acquired a chromosome segment substitution line CSSL 9311 that carries a 13 Mb genome segment containing OsMYB8 from the donor parent 9311 (an indica variety) in the japonica variety XiuShui134 (XS134) background [29] . Under field conditions, NIL TFB and CSSL 9311 plants exhibited about 0.5 h earlier DFOT than their recurrent parents (Fig. 7a, b, d, e ), without obvious impacts on the tiller number, plant height, heading date, panicle traits, and seed setting rate (Supplementary Fig. 15 ). In addition, RT-qPCR results showed that the expression levels of OsMYB8 and OsJAR1 in NIL TFB and CSSL 9311 lodicules were higher than that in ZH11 and XS134, respectively (Fig. 7c, f ). Therefore, the OsMYB8 Hap1 allele could promote floret opening in japonica varieties, conferring great potential to improve japonica DFOT and hybrid seed production. Fig. 7: The indica allele of OsMYB8 promotes japonica DFOT. a , d Comparison of panicles in ZH11 and NIL TFB ( a ) XS134 and CSSL 9311 ( d ) at 12:00 noon in October 2022 in Guangzhou. Scale bars, 1 cm. b , e Number of opened florets in ZH11 and NIL TFB ( b ) XS134 and CSSL 9311 ( e ) at different time points of the day in October 2022 in Guangzhou. Values are mean ± SEM. ( n = 10 panicles). c , f Relative expression levels of OsMYB8 and OsJAR1 in lodicules of ZH11 and NIL TFB ( c ) XS134 and CSSL 9311 ( f ). Values are mean ± SEM. ( n = 3 biological replicates). Significance is evaluated by the two-sided Student’s t -test, and P values are indicated. g A model depicting an OsMYB8 - OsJAR1 module regulating differential DFOT in indica and japonica rice. Natural variation in the promoter sequences of OsMYB8 confers higher expression level of OsMYB8 in indica , thus higher accumulation of JA-Ile and earlier DFOT in indica as compared to japonica . Source data are provided as a Source Data file. Full size image Indica and japonica are two subspecies of Asian cultivated rice domesticated from the wild rice O. rufipogon [28] . Due to long-term adaptation to different ecological niches, indica and japonica rice have evolved to exhibit a differentiated DFOT, which might be beneficial for promoting prezygotic reproductive isolation by preventing mating and hybridization, thus facilitating divergence of these two subspecies. However, the asynchronized DFOT of the indica and japonica parental lines hindered the utilization of the strong heterosis of indica - japonica hybrid rice. DFOT is a complex quantitative trait and is easily affected by environmental factors (such as light, temperature and humidity) [30] , [31] , [32] , [33] . Although a number of quantitative trait loci (QTL) for DFOT has been previously mapped to different chromosomes of rice, none of them has been molecularly cloned, largely due to the difficulty in precise phenotyping and the small additive effects of the individual locus (typically less than 10% phenotypic variance) [34] , [35] , [36] , [37] , [38] . In this study, we identified OsMYB8 as a key regulator of DFOT in both indica and japonica rice through comprehensive comparative, time-course transcriptome analyses of the lodicules of a representative indica TFB and a representative japonica ZH11. We showed that expression of OsMYB8 is up-regulated in the lodicules before floret opening and reaches a plateau at the peak opening time, then gradually declines (Fig. 2d , Supplementary Fig. 5 ). We further identified OsJAR1 as a direct target gene of OsMYB8 , which acts to promote the conversion of JA into biologically active JA-IIe and regulate the expression of genes related to cell osmolality and cell wall remodeling in the lodicules, thus promoting floret opening. Strikingly, we demonstrated that natural variation (6 SNPs) in the 2-kb promoter region of OsMYB8 confers higher expression of OsMYB8 , and thus higher expression of OsJAR1 and higher accumulation of JA-IIe in lodicule cells, ultimately leading to earlier DFOT in indica rice compared to japonica rice (Fig. 7g ). Thus, our results provided insights into the genetic and molecular regulation of DFOT in rice. Previous studies have documented ample evidence that jasmonate is a vital hormone regulating multiple reproductive processes including flower opening time, and stamen/female organ development, and fertility [39] , [40] . MYB transcription factors, especially R2R3-MYB members, have been shown to function as key regulators in JA-mediated flower opening and floral organ development in different plant species [41] , [42] . For example, AtMYB21/24, two homologs of OsMYB8, are targets of JAZ repressors and could interact with MYC2/3/4/5 to regulate petal elongation (thus leading to petal opening), stamen development, and pollen fertility in Arabidopsis [43] , [44] . The tomato homolog SlMYB21 regulates floret opening as well as carpel and ovule development, through promoting JA biosynthesis in a positive-feedback manner [45] . Previous studies have also reported that the rice mutants deficient in JA biosynthesis and signaling, such as allene oxide cyclase ( Osaoc ), oxophytodienoate reductase 7 ( Osopr7 ), jasmonate resistant 1 ( Osjar1 ) and coronatine insensitive ( Oscoi1a, Oscoi1b and Oscoi2 ) mutants, usually exhibit defects in spikelet morphology, anther dehiscence, flower opening and spikelet fertility [46] , [47] , [48] , [49] . In this study, we showed that OsMYB8 acts upstream of OsJAR1 to promote JA synthesis, and the Osmyb8 mutant exhibits delayed DFOT, but normal spikelet morphology, pollen maturation, and fertility (Supplementary Fig. 7 ), suggesting that OsMYB8 mainly functions in controlling the floret opening time, and it represents an elite gene resource for improving DFOT in rice, with minimal negative pleiotropic effect on stamen development. Notably, phylogenetic analysis identified an OsMYB8-like gene in the rice genome that shares 45.2% homology with OsMYB8 (Supplementary Fig. 3 , Supplementary Fig. 16a ), and it was preferentially expressed in stamen (Supplementary Fig. 16b ), hinting a possible role in regulating stamen development. Further studies are required to elucidate the biological function of the OsMYB8-like gene in the future. Earlier studies have shown that the lodicule undergoes dramatic changes in multiple physiological processes during floret opening and closure, including an increase in soluble sugar content, which leads to a rise in cell osmotic pressure to drive water uptake by the lodicules [13] . An earlier study has demonstrated a critical role of auxin signaling cascade in regulating floret opening. The authors demonstrated that OsARF2 and OsARF18 antagonistically regulate the expression of OsSUT1 (a sucrose transporter gene) to regulate sucrose transport from the source tissues (vegetative organs) into the sink tissues (reproductive organs) and floret opening [50] . It will be worthy to investigate how the OsMYB8 -mediated JA signaling pathway cross-talks with the auxin signaling pathway to coordinately regulate DFOT in future studies. In addition, recent studies have demonstrated that DFOT1/EMF1 negatively regulate DFOT through modulating the activity of pectin methylesterases (PMEs), thus loosening the stiffness of cell walls of lodicules cells [11] , [20] . In this study, our transcriptome and RT-qPCR analyses indicated that OsMYB8 regulates the expression levels of various genes related to the cell wall modification. In addition, we also observed that the expression of these genes was altered in the lodicules of the Osjar1 mutants. Thus, we speculate that OsMYB8-OsJAR1 module likely regulates floret opening through regulating cell wall relaxation and expansion. It is also worth noting that DFOT is easily affected by environmental factors, such as light, temperature, and humidity [30] , [31] , [32] , [33] . We found that the OsMYB8 promoters of japonica and indica varieties contain various cis-elements responsive to light, temperature, and hormones based on sequence analysis with PLANTCARE . How these external factors influence the expression of OsMYB8 , and thus DFOT will be an interesting avenue for future research. Inter-subspecific indica-japonica hybrid rice was proposed to be an important direction of future rice breeding due to its superior heterosis. Nevertheless, current breeding and utilization of indica - japonica hybrid rice is still hampered by asynchronized DFOT (and thus low yield of hybrid seed production) in the indica and japonica parental lines. In this study, we showed that elevating expression level of OsMYB8 in the japonica background or introgression of the Hap1 allele of OsMYB8 from indica varieties into japonica varieties could promote DFOT over half an hour, thus effectively reducing the interval between the DFOT of indica and japonica varieties (Fig. 7a, b, d, e ). Importantly, we did not find any significant negative impact of the introgression of OsMYB8 Hap1 allele on other agronomic traits (plant architecture and heading date, Supplementary Fig. 14 ). Thus, further manipulation of OsMYB8 expression levels may offer a feasible approach to facilitate hybrid seed production and utilization of inter-subspecific indica - japonica hybrid rice. Plant materials and growth conditions Rice cultivar ZhongHua11 (ZH11) ( Oryza sativa cv. Japonica ) and TianFengB (TFB) ( Oryza sativa cv. Indica ) were used as wild-type controls for mutation or transgenic analyses. The 529 core rice germplasm resources were supplied by National Key Laboratory of Crop Genetic Improvement, Huazhong Agricultural University [26] (Supplementary Data 8 ). A total of 40 elite rice varieties, including 12 japonica varieties and 28 indica varieties, were kindly supplied by D. Zhou and were used for DFOT investigation (Supplementary Data 1 ). XiuShui134 (XS134) and the CSSL line carrying OsMYB8 9311 were kindly provided by B. Hu and C. Chu. For NIL TFB construction, F 1 of ZH11 and TFB plants were backcrossed with ZH11, and NIL TFB were selected in the BC 4 F 3 generation with molecular markers. All rice plants were grown in the experimental field of the South China Agricultural University in Guangzhou (23°7’ N, 113°15’ E) from March to November in 2019 to 2023, and in Lingshui, Hainan (18°22’ N, 109°45’ E) from November to April in 2019 to 2023. Transgene construct preparation and rice transformation To generate the Osmyb8 and Osjar1 knockout lines, gene-specific guide RNA sequences were designed with an online software toolkit CRISPR-GE [51] and cloned into the CRISPR/Cas9 binary vector pYLCRISPR/Cas9Pubi-H [52] . To generate the OsMYB8 TF /ZH11 and OsMYB8 TF / Osmyb8 ZH transgenic lines, the OsMYB8 genomic fragment (including 2-kb promoter, coding region, and 1.5 kb 3′UTR) was amplified from TFB gDNA and inserted into the pCAMBIA1300 vector, forming a recombinant plasmid p1300-OsMYB8 . To generate the proOsMYB8::GUS construct, the 2-kb promoter sequence of OsMYB8 was amplified from TFB gDNA and cloned into pCAMBIA1305.1 for plant transformation. To construct the proOsMYB8::JAR1 plasmid, the OsJAR1 coding sequence was amplified from ZH11 cDNA and cloned into the pCAMBIA1300 vector driven by the 2-kb promoter sequence of OsMYB8 from TFB gDNA. To generate the proOsMYB8::OsMYB8-GFP construct, the OsMYB8 coding sequence (without stop codon) was amplified from ZH11 cDNA and cloned into the pOx - eGFP vector driven by the 2-kb promoter sequence of OsMYB8 from TFB gDNA. The above constructs were transformed into indicated background by Agrobacterium-mediated transformation (Biogle Biological Company, China). Hygromycin (hyg) was used for screening the positive transgenic lines. The mutation sites or gene expression levels were examined by DNA sequencing or RT-qPCR analysis. The primers used for vector constructions are listed in Supplementary Data 11 . Measurement of the water content in lodicules 100 pairs of lodicules were carefully extracted from the florets and collected as one sample. The fresh weight of each sample was firstly measured using an analytical balance. Then, the samples were dried at 65 °C overnight, and the dry weight of each sample was measured again. The water content of the lodicules was determined by subtracting the dry weight from the fresh weight. Three biological replicates were performed for each sample. RNA extraction and RT-qPCR analysis Total RNAs were extracted from lodicules and other tissues using TRIzol reagent (Thermo Fisher, USA). The complementary DNAs (cDNAs) were synthesized by reverse-transcription according to the manufacturer’s instructions (Yeasen, China). RT-qPCR was performed using the LightCycler96 real-time PCR system (Roche, Switzerland) with the qPCR SYBR Green Master Mix (Yeasen, China) according to the manufacturer’s instructions. The OsActin1 gene ( LOC_Os03g50885 ) was used as the internal control. The expression level of genes was calculated using the 2 -ΔCt method. All the primers used for RT-qPCR above are shown in Supplementary Data 11 . RNA-seq analysis The lodicules of rice were separated by tweezers and were frozen immediately in liquid nitrogen for RNA-seq analysis. Three biological replicates were performed for each sample, except for the samples of TF with two biological replicates. RNA sequencing was performed at the Azenta company using the Illumina Hiseq platform. For data analysis, the processed reads were compared with Hisat2 v2.0.1 [53] to the reference genome MSU Release 7.0 [54] . HTSeq v0.6.1 [55] was used for quantitative analysis of genes. DESeq2 [56] was used for differential expression analysis, and P -value < 0.05, absolute log 2 FC ≥ 1 were used for screening of the differentially expressed genes. The Gene Ontology (GO) analysis was conducted with the David database ( https://david.ncifcrf.gov/home ). GUS staining and histological observation For histochemical analysis, the florets about 1–2 h before opening from proOsMYB8::GUS transgenic lines were collected for staining using the GUS stain Kit (Coolaber, China) according to the manufacturer’s protocol. After staining, the florets were decolorized with 70% (v/v) ethanol and photographed under a Zeiss dissecting microscope. Subcellular localization To determine the subcellular localization of OsMYB8, the coding sequence of OsMYB8 without the stop codon was amplified from cDNA of the ZH11 and cloned into the pCAMBIA1305-35S::GFP vector, resulting in the 35 S::OsMYB8-GFP construct. The nuclear-localized protein D53 fused with mCherry was used as a nuclear marker [57] . The 35 S::OsMYB8-GFP and p35S::D53-mCherry fusion constructs were transiently co-transformed into rice protoplasts. The GFP and mCherry fluorescence in protoplasts were observed with a confocal microscope (Zeiss LSM780, Germany). Droplet digital PCR Droplet digital PCR (ddPCR) was performed to select single copy transgene of OsMYB8 TF in the Osmyb8 ZH background [58] . The ddPCR reaction mixture consists of 10 μL of 2 × ddPCR super mix for probes (Bio-Rad, USA), 50~100 ng DNA, 900 nM OsMYB8 primers/250 nM probe (5′ FAM, 3′ BHQ1), 900 nM OsActin1 primers/250 nM probe (5′ HEX, 3′ BHQ1) and variable ddH 2 O in a final volume of 20 μL. The entire reaction mixture was loaded into a disposable plastic cartridge (Bio-Rad, USA) together with 60 μL of droplet generation oil (Bio-Rad, USA) and placed into the droplet generator (Bio-Rad, USA). After processing, the droplets generated from each sample were transferred to a 96-well PCR plate (Eppendorf, Germany). PCR amplification was carried out on a T100 Touch thermal cycler (Bio-Rad, USA) using a thermal profile beginning at 95 °C for 10 min, followed by 45 cycles of 94 °C for 10 s, and 58 °C for 60 s, and ending of 98 °C for 10 min at a ramp rate of 2 °C/s. After PCR, the plate was loaded on the droplet reader (Bio-Rad, USA). The Data were analyzed using the QuantaSoft Analysis Pro software (Bio-Rad, USA). DAP-seq analysis DAP-seq (DNA affinity purification sequencing) is a method used to identify DNA-binding sites of transcription factors [59] . Briefly, 10 μg of ZH11 genomic DNA was broken into 200-bp fragments, fragmented gDNA were constructed into libraries using the VAHTS Universal Pro DNA Library Prep Kit for Illumina (Vazyme, China). The coding sequence of OsMYB8 was cloned into the pGEX-4T1 vector to generate the GST-OsMYB8 recombinant construct. GST-OsMYB8 recombinant protein or GST protein were purified from E.coli strain (DE3) with Glutathinone Sepharose Beads (Sangon, China). The production of GST-OsMYB8 recombinant protein was induced by the addition of 0.4 mM isopropyl b-D-thiogalactopyranoside and grown at 16 °C overnight, and then were purified with GST 4FF Sefinose (TM) Resin Kit (Sangon Biotech, China) according to the manufacturer’s protocol. The purified protein was incubated with 500 ng adaptor-ligated gDNA library at room temperature for 2 h before washing away the unbound DNA fragments. The GST proteins were used as the controls. The eluted DNAs were then sequenced using the Illumina HiSeq sequencing platform with two technical replicates. The clean reads were aligned to the reference genome MSU Release 7.0 using Bowtie2 v2.3.5.1 [60] . Aligned reads were sorted and duplicated reads were removed by SAMtools v1.12 [61] . Peaks were called using MACS2 v2.1.0 [62] ( P < 0.01). Peaks were identified using the MEME-ChIP online software ( https://meme-suite.org/meme/ ). Putative genes associated with peaks were annotated using ChIPseeker v1.32.1 [63] . Yeast two-hybrid assay For Y2H assay, the full-length or truncated CDS of OsMYB8 were amplified and cloned into the vector pGBKT7 , and then the recombinant plasmid and pGADT7 were co-transformed into AH109 yeast cells mediated by PEG4000. The positive transformants were first selected on the (SD)/-Leu/-Trp medium and then transferred to (SD)/-His/-Leu/-Trp and (SD)/-Ade/-His/-Leu/-Trp selection medium (Coolaber, China). The empty vector pGBKT7 and pGADT7 were co-transformed as negative controls. Electrophoretic mobility shift assay Native and mutated probes were synthesized and labeled with biotin using the electrophoretic mobility shift assay (EMSA) Probe Biotin Labeling Kit (Beyotime, China). EMSAs were carried out using a Chemiluminescent EMSA Kit (Beyotime, China). Briefly, biotin-labeled probes were incubated for 20 min with the GST or GST-OsMYB8 protein in the binding buffer at room temperature. For competition reaction, 5× and 20× unlabeled cold probes were mixed with the labeled probes. The DNA-protein complex was separated by 5% native polyacrylamide gel electrophoresis and the signal of biotin was photographed using the Biostep Celvin S420 system (Biostep, German). The probes used in this study are listed in Supplementary Data 11 . Transient transcription dual-LUC assay For dual-LUC assay, the ~2-kb OsJAR1 promoter was amplified and inserted into the pGreenII0800-LUC vector to generate the reporter plasmid. The OsMYB8 coding sequence without stop codon was amplified and inserted into the pUC19 vector to generate the effector plasmid. The effector and reporter plasmids were co-transformed into rice protoplasts and incubated in darkness at 28 °C for 12 h. The protoplasts were collected and disintegrated in passive lysis buffer provided in Dual-Luciferase Reporter Gene Assay Kit (Yeasen, 11402ES60). Luciferase activity was also measured using GloMax2020 (Promega) following the manufacturer’s instructions. Renilla luciferase (REN) driven by 35S promoter in pGreenII0800-LUC was used as the internal control. The relative firefly luciferase activity was counted as the ratio of LUC/REN for each sample. Chromatin immunoprecipitation assay For ChIP assays, rice florets of the ZH11 and transgenic pOsMYB8::OsMYB8-GFP plants were harvested and cross-linked in a fixation buffer with 1% (v/v) formaldehyde under vacuum for 20 min. Glycine was added to terminate the cross-linking reaction. The prepared chromatin complexes were sonicated into 200–500 bp fragments and then precleared with protein A magnetic beads (Merck Millipore, USA) [64] . For immunoprecipitations, Anti-GFP (Nanobody) Magnetic beads (ABclonal, China) were added into samples and incubated overnight at 4 °C. DNA was precipitated with magnetic beads. For the real-time-qPCR reaction, the precipitated DNA was recovered and dissolved in water as the template. The enrichment was standardized to the input DNA to obtain the fold enrichment. An unrelated DNA sequence from the rice OsActin1 gene was used as an internal control. All relevant primers used in the ChIP assay are listed in Supplementary Data 11 . Measurement of JA-Ile concentration The quantification of JA-Ile was conducted by Wuhan Metware Biotechnology Co., Ltd, located in Wuhan, China. Approximately 50 mg of lodicules sample was frozen in liquid nitrogen and ground into a fine powder. The sample extracts were analyzed using an LC-ESI-MS/MS system (HPLC: Shim-pack UFLC SHI-MADZU CBM30A system; Shimadzu MS, Applied Biosystems 6500 Triple Quadrupole). The analytical conditions of HPLC were as follows, LC: column, Waters ACQUITY UPLC HSS T3 C18 (100 mm × 2.1 mm, 1.8 µm); solvent system, water with 0.04% acetic acid (A), acetonitrile with 0.04% acetic acid (B); gradient program, started at 5% B (0–1 min), increased to 95% B (1–8 min), 95% B (8–9 min), finally ramped back to 5% B (9.1–12 min); flow rate, 0.35 mL/min; temperature, 40 °C; injection volume: 2 μL. The ESI source operation parameters were as follows: ion source, ESI ±; source temperature 550 °C; ion spray voltage (IS) 5.5 kV (positive), −4.5 kV (negative); curtain gas (CUR) was set at 35 psi, respectively. The contents of JA-Ile were determined using an internal standard method, with three biological replications performed for each sample. Measurement of sugar concentration The quantification of sugar in the lodicules was conducted by Wuhan Metware Biotechnology Co., Ltd, Wuhan, China. The freeze-dried materials were crushed using a mixer mill (MM 400, Retsch) with a zirconia bead for 1.5 min at 30 Hz. 20 mg of powder was diluted to 500 μL with methanol: isopropanol: water (3:3:2 V/V/V), vortexed for 3 min and ultrasound for 30 min. The extract was centrifuged at 13,188 × g under 4 °C for 3 min. 50 μL of the supernatant was mixed with 20 μL internal standard (ribitol, 100 μg/mL) and evaporated under nitrogen gas stream. The evaporated sample was transferred to the lyophilizer for freeze-drying. The residue was used for further derivatization. The derivatization method was as follows: the sample was mixed with 100 μL solution of methoxyamine hydrochloride in pyridine (15 mg/mL). The mixture was incubated at 37 °C for 2 h. Then 100 μL of BSTFA was added into the mixture and kept at 37 °C for 30 min after vortex-mixing. The mixture was analyzed using GC-MS after being diluted to an appropriate concentration. Agilent 7890B gas chromatograph coupled to a 7000 D mass spectrometer with a DB-5MS column (30 m length × 0.25 mm i.d. × 0.25 μm film thickness, J&W Scientific, USA) was employed for GC-MS analysis of sugars. Helium was used as carrier gas, at a flow rate of 1 mL/min. Injections were made in the split mode with a split ratio 3:1 and the injection volume was 3 μL. The oven temperature was held at 170 °C for 2 min, and then raised to 240 °C at 10 °C/min, raised to 280 °C at 5 °C/min, raised to 310 °C at 25 °C/min, and held at the temperature for 4 min. All samples were analyzed in selective ion monitoring mode. The ion source and transfer line temperature were 230 °C and 240 °C, respectively. Three biological replicates were performed for each sample. Phylogenetic analysis of R2R3-MYB transcription factors There are 89 and 124 R2R3-MYB transcription factors in rice and Arabidopsis respectively [65] . The full-length protein sequences of R2R3-MYB transcription factors from both the rice and Aarabidopsis genomes were obtained from Ensembl database ( http://plants.ensembl.org/index.html ). These sequences were then aligned using ClustalW in MEGA7 [66] . A neighbor-joining phylogenetic tree was constructed based on the alignment, using the poisson correction method and pairwise deletion of gaps. The reliability of the tree was assessed by bootstrap analysis with 1000 replicates. Haplotype analysis The 2-kb promoter sequence of OsMYB8 in 3513 cultivated rice accessions were retrieved from the RiceVarMap2.0 database ( http://ricevarmap.ncpgr.cn/v2/ ), and haplotype analysis was carried out using the method in the database. Only haplotypes found in ≥ 10 rice accessions were recorded. Nucleotide diversity and fixation index calculation The raw sequencing data of the 386 cultivated rice were downloaded from NCBI with BioProject PRJNA171289 (>2.5× per genome) [26] . The raw sequencing data of the 185 wild rice were downloaded from NCBI with BioProject accession number PRJNA658215 (>5× per genome) [27] . We mapped the reads to the reference genome MSU Release 7.0 using BWA v0.7.12 [67] , sorted and indexed the resulting BAM files using SAMtools v1.12 [61] . 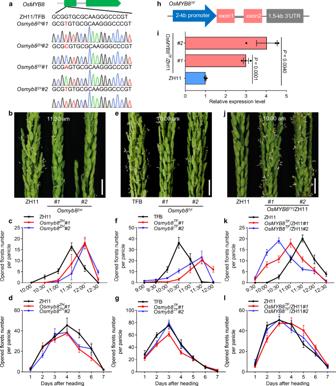Fig. 3:OsMYB8positively regulates rice DFOT. aCreation of theOsmyb8mutants using the CRISPR/Cas9 genome editing approach.Osmyb8mutants in ZH11 and TFB backgrounds were named asOsmyb8ZHandOsmyb8TFrespectively. The upper panel shows a schematic diagram of theOsMYB8gene bearing the CRISPR/Cas9 target site. The mutation site was indicated in red.b,e,jComparison of panicles in ZH11 andOsmyb8ZHmutants at 11:30 am (b) TFB andOsmyb8TFmutants at 10:00 am (e) ZH11 andOsMYB8TF/ZH11 lines at 10:00 am in June 2021 in Guangzhou (j). Scale bars, 1 cm.c,f,kNumber of opened florets per panicle in ZH11 andOsmyb8ZHmutants (c), TFB andOsmyb8TFmutants (f), and ZH11 andOsMYB8TF/ZH11 lines (k) at different time points of the day in June 2021 in Guangzhou. Values are means ± SEM. (n= 8 panicles).d,g,lNumber of opened florets in ZH11 andOsmyb8ZHmutants (d), TFB andOsmyb8TFmutants (g), and ZH11 andOsMYB8TF/ZH11 lines (l) at different days after heading in June 2021 in Guangzhou. Values are means ± SEM. (n= 10 panicles).hSchematic diagram of the vector structure used for constructingOsMYB8TF/ZH11 transgenic plants.iRT-qPCR analysis ofOsMYB8transcripts levels in the lodicules of theOsMYB8TF/ZH11 transgenic lines. ZH11 was used as a negative control. Values are means ± SEM. (n= 3 biological replicates). Significance is evaluated by the two-sided Student’st-test, andPvalues are indicated. Source data are provided as a Source Data file. The SNPs were identified using GATK v4.2.0.0 [68] , the GVCFs of each sample were generated with HaplotypeCaller. We then used CombineGVCFs and GenotypeGVCFs to generate VCF file, the variations were further filtered by VariantFiltration. Nucleotide diversity (π) and fixation index (F ST ) of OsMYB8 in wild rice and cultivated rice were calculated using VCFtools v0.1.16 [69] with 20-kb windows and 2-kb steps on the 100-kb region. Statistical analysis We used GraphPad Prism 8 for statistical analysis. Data are mean ± SEM. 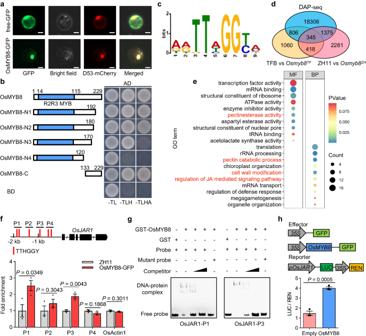Fig. 4: Identification of the genome-wide direct targets of OsMYB8. aNuclear localization of OsMYB8-GFP in rice protoplasts. D53-mCherry was used as a nuclear marker. Scale bars, 20 μm.bYeast two-hybrid assay showing the transcriptional activity of OsMYB8. Left is the diagrams of full-length and truncated OsMYB8 proteins, which were fused with the DNA-binding domain (BD).cThe core binding motif of OsMYB8 protein identified using MEME-ChIP.dVenn diagrams showing a comparison of DAP-seq binding genes with the identified DEGs inOsmyb8mutants by RNA-seq.eGO enrichment analysis of 345 overlap genes in (d). MF indicates molecular function, BP indicates biological process.fChIP-qPCR analysis showing that OsMYB8 binds to theOsJAR1promoter in vivo. The upper panel is a diagram ofOsJAR1promoter with the indicated regions used for detection by ChIP-qPCR. The red lines indicate the position of “TTHGGY” motifs in theOsJAR1promoter regions. Immunoprecipitation was performed with anti-GFP antibody, ZH11 was used as a negative control. (n= 3 technical replicates).gEMSA assay showing that GST-OsMYB8 recombinant protein directly binds to the “TTHGGY” motif-containing regions of theOsJAR1promoter. Unlabeled probes were used as competitors. GST was used as a negative control.hTransient dual-LUC assay showing that OsMYB8 induces the transcriptions ofOsJAR1promoter in rice protoplasts. The upper panel is diagrams of various constructs used in the transient expression assay. The expression level of REN was used as an internal control. The LUC/REN ratio represents the relative activity of theOsJAR1promoter. (n= 3 technical replicates). The Values in (f) and (h) are means ± SEM. Significance is evaluated by the two-sided Student’st-test, andPvalues are indicated. The subcellular localization experiments in (a) and the EMSA experiments in (g) were independently repeated three times with similar results. Source data are provided as a Source Data file. 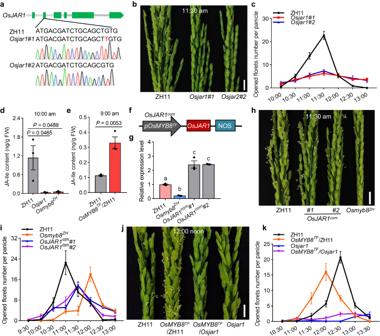Fig. 5:OsJAR1influences JA-Ile content in lodicule to regulate rice DFOT. aCreation of theOsjar1mutants in ZH11 background using the CRISPR/Cas9 genome editing approach. The mutation site was indicated in red.bComparison of panicles in ZH11 andOsjar1mutants at 11:30 am in June 2022 in Guangzhou. Scale bars, 1 cm.cNumber of opened florets per panicle in ZH11 andOsjar1mutants at different time points of the day. Values are mean ± SEM. (n= 10 panicles).d,eJA-Ile content in lodicules at 10:00 am of ZH11,Osjar1,andOsmyb8ZH(d) at 9:00 am of ZH11 andOsMYB8TF/ZH11(e). Values are mean ± SEM. (n=  3 biological replicates). Significance is evaluated by the two-sided Student’st-test, andPvalues are indicated.fSchematic diagram of the vector structure used for constructingOsJAR1commaterials. ThepOsMYB8TFmeans the promoter was amplified from TFB.gRelative expression level ofOsJAR1in the lodicules of ZH11,OsJAR1comandOsmyb8ZH. Values are means ± SEM. (n= 3 biological replicates). Letters above the bars indicate significant differences (P< 0.05), as evaluated by one-way ANOVA with Tukey’s multiple comparisons test.h,jComparison of panicles in ZH11,OsJAR1comandOsmyb8ZHat 11:30 am in June 2022 in Guangzhou (h) and in ZH11,OsMYB8TF/ZH11,OsMYB8TF/Osjar1andOsjar1at 12:00 noon in October 2022 in Guangzhou (j). Scale bars, 1 cm.iNumber of opened florets in ZH11,OsJAR1com,andOsmyb8ZHat different time points of the day in June 2022 in Guangzhou. Values are mean ± SEM. (n= 10 panicles).kNumber of opened florets in ZH11,OsMYB8TF/ZH11,OsMYB8TF/Osjar1,andOsjar1at different time points of the day in October 2022 in Guangzhou. Values are mean ± SEM. (n= 10 panicles). Source data are provided as a Source Data file. 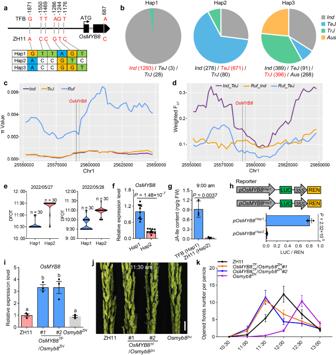Fig. 6: Natural variation inOsMYB8promoter confers DFOT divergence injaponicaandindica. aHaplotype analysis ofOsMYB8promoter in the 3513 rice germplasms. Nucleotide variations in the 2-kb promoter ofOsMYB8were shown.bDistribution frequency of the threeOsMYB8haplotypes in diverse Asian cultivated rice accession. The haplotype with the largest number was highlighted in red.cNucleotide diversity (π) of a 100-kb genomic region surroundingOsMYB8in theindica(Ind),temperate japonica(TeJ) andO. rufipogon(Ruf). The regions (Chr1: 25,590,725–25,592,725) between two black vertical lines indicates the position ofOsMYB8promoter.dFSTvalues ofTeJ_Ind,Ruf_TeJ, andRuf_Indin a 100-kb genomic region surroundingOsMYB8. The region (Chr1: 25,590,725–25,592,725) between two black vertical lines indicates the position ofOsMYB8promoter.eThe DFOT of the rice accessions with Hap1 and Hap2 in May 2022 in Guangzhou. (n= 30 accessions).fRelative expression levels ofOsMYB8in lodicules of the rice accessions with Hap1 and Hap2, respectively. (n= 10 accessions).gJA-Ile content in TFB and ZH11 lodicules at 9:00 am. (n= 3 biological replicates).hTransient dual-luciferase assays showing the transcriptional activity ofpOsMYB8Hap1andpOsMYB8Hap2in rice protoplasts. (n= 3 technical replicates). The values inf–hare shown as mean ± SEM. Significance is evaluated by the two-sided Student’st-test, andPvalues are indicated.iRelative expression levels ofOsMYB8in lodicules of ZH11,OsMYB8TF/Osmyb8ZHtransgenic lines and theOsmyb8ZHmutant. Values are mean ± SEM. (n= 3 biological replicates). Letters above the bars indicate significant differences (P< 0.05), as evaluated by one-way ANOVA with Tukey’s multiple comparisons test.jComparison of panicles in ZH11,OsMYB8TF/Osmyb8ZHtransgenic lines and theOsmyb8ZHmutant at 11:30 am in October 2022 in Guangzhou. Scale bars, 1 cm.kNumber of opened florets in ZH11,OsMYB8TF/Osmyb8ZHtransgenic lines, and theOsmyb8ZHmutant at different time points of the day in October 2022 in Guangzhou. Values are mean ± SEM. (n= 10 panicles). Source data are provided as a Source Data file. 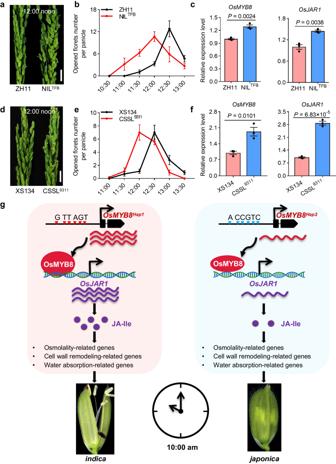Fig. 7: Theindicaallele ofOsMYB8promotesjaponicaDFOT. a,dComparison of panicles in ZH11 and NILTFB(a) XS134 and CSSL9311(d) at 12:00 noon in October 2022 in Guangzhou. Scale bars, 1 cm.b,eNumber of opened florets in ZH11 and NILTFB(b) XS134 and CSSL9311(e) at different time points of the day in October 2022 in Guangzhou. Values are mean ± SEM. (n= 10 panicles).c,fRelative expression levels ofOsMYB8andOsJAR1in lodicules of ZH11 and NILTFB(c) XS134 and CSSL9311(f). Values are mean ± SEM. (n= 3 biological replicates). Significance is evaluated by the two-sided Student’st-test, andPvalues are indicated.gA model depicting anOsMYB8-OsJAR1module regulating differential DFOT inindicaandjaponicarice. Natural variation in the promoter sequences ofOsMYB8confers higher expression level ofOsMYB8inindica, thus higher accumulation of JA-Ile and earlier DFOT inindicaas compared tojaponica. Source data are provided as a Source Data file. Two-sided unpaired Student’s t -test was used to test the significant difference between two groups. Three groups and more were analyzed by one-way analysis of variance (ANOVA) with Tukey’s multiple comparisons test. Reporting summary Further information on research design is available in the Nature Portfolio Reporting Summary linked to this article.